Pure and stable metallic phase molybdenum disulfide nanosheets for hydrogen evolution reaction Metallic-phase MoS 2 (M-MoS 2 ) is metastable and does not exist in nature. Pure and stable M-MoS 2 has not been previously prepared by chemical synthesis, to the best of our knowledge. Here we report a hydrothermal process for synthesizing stable two-dimensional M-MoS 2 nanosheets in water. The metal–metal Raman stretching mode at 146 cm −1 in the M-MoS 2 structure, as predicted by theoretical calculations, is experimentally observed. The stability of the M-MoS 2 is associated with the adsorption of a monolayer of water molecules on both sides of the nanosheets, which reduce restacking and prevent aggregation in water. The obtained M-MoS 2 exhibits excellent stability in water and superior activity for the hydrogen evolution reaction, with a current density of 10 mA cm −2 at a low potential of −175 mV and a Tafel slope of 41 mV per decade. The metallic-phase MoS 2 (M-MoS 2 ) is a single-layer S-Mo-S structure in which each molybdenum atom is surrounded by six sulfur atoms in an octahedral lattice. With dense active sites and an electronic conductivity that is six orders of magnitude higher than that of the semiconductor phase of MoS 2 (S-MoS 2 ) (ref. 1 ), M-MoS 2 has emerged as a promising candidate for a broad range of applications and is expected to exhibit better performance than its semiconducting counterpart, in particular in the hydrogen evolution reaction (HER) and as a photocatalyst and supercapacitor [2] , [3] , [4] , [5] . These attractive properties of M-MoS 2 are offset by the fact that a pure phase of M-MoS 2 is very challenging to prepare, because it is highly unstable. Over the past few decades, many efforts to develop a process to prepare stable and highly pure M-MoS 2 have largely proved futile. A complicated method for the preparation of metastable M-MoS 2 using lithium intercalation of S-MoS 2 has been reported [5] , [6] , [7] , [8] . However, the reported M-MoS 2 suffered from coexistence with S-MoS 2 in a relative proportion of 50–80% (refs 3 , 9 ). In addition, the intermediary Li x MoS 2 and intercalator of n-butyllithium are both dangerous materials that may self-heat [8] and are highly pyrophoric in air [5] . The preparation procedures are also tedious and can take as long as 3 days [10] , [11] . The previously mentioned M-MoS 2 easily transformed to S-MoS 2 due to S–S van der Waals interactions [12] , [13] , [14] . Therefore, an efficient synthesis method for the production of a large quantity of stable and pure M-MoS 2 is still highly desirable. M-MoS 2 could be an intermediary state during the synthesis of S-MoS 2 , which is a stable form in many chemical reactions [15] , [16] . This approach provides a possible method for capturing the metastable M-MoS 2 even though it is thermodynamically unstable and may rapidly transform to S-MoS 2 at elevated temperatures. In fact, S-MoS 2 can transform into an octahedral structure of M-MoS 2 under a high pressure of 35 GPa (refs 17 , 18 , 19 ), which implies that the metallic phase of MoS 2 may be achievable at a relatively low temperature, a specific pressure and a proper chemical environment. Therefore, we employ octahedral MoO 3 as the starting material in a pressurized hydrothermal process, to directly grow highly pure M-MoS 2 in water. The as-prepared M-MoS 2 is highly stable in water due to the reduced stacking of the layered materials, which are separated by water molecules. Urea, which is a weak reducing agent, plays a key role in the formation of M-MoS 2 . The structure of octahedral MoO 3 can be maintained under acidic conditions. To satisfy the expected growth conditions, thioacetamide is chosen as the sulfur source and the reaction is maintained at a low pH value (pH ∼ 4). The synthesis of M-MoS 2 is performed at 200 °C by mixing MoO 3 , thioacetamide and urea in an autoclave. The as-prepared M-MoS 2 is pure and stable with high activity for the HER. 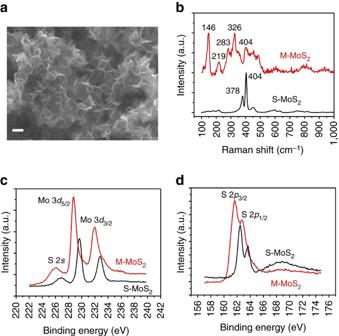Figure 1: Morphology of M-MoS2and phase identification of M-MoS2and S-MoS2. (a) SEM image of M-MoS2showing the nanosheet structures. Scale bar, 100 nm. (b) Raman shift of M-MoS2and S-MoS2. (c,d) High-resolution X-ray photoelectron spectroscopy (XPS) spectra of Mo 3d(c) and S 2p(d) for M-MoS2and S-MoS2. Highly pure metallic phase MoS 2 Figure 1a shows a typical scanning electron microscopic (SEM) image of the as-prepared M-MoS 2 sample. The MoS 2 nanosheets are 100 nm in size and a few nanometres in thickness. The morphology of S-MoS 2 is similar to that of M-MoS 2 on the nanoscale ( Supplementary Fig. 1 ). The results from energy dispersive X-ray spectroscopy indicated that the S to Mo atomic ratio of the as-prepared M-MoS 2 is ∼ 2.05 ( Supplementary Fig. 2 ). The most notable difference between M-MoS 2 and S-MoS 2 is the symmetry of the sulfur in their structures. The structural variations result in significant differences in their characteristic Raman features. Figure 1b shows the Raman spectra of M-MoS 2 and S-MoS 2 synthesized at 200 °C and 240 °C, respectively. A strong Raman band is observed at 146 cm −1 and attributed to Mo–Mo stretching vibrations in M-MoS 2 . Calculations have predicted this band at the K points of the Brillouin zone for octahedrally coordinated distorted MoS 2 (ref. 12 ). Our results confirm the existence of this band in M-MoS 2 . The Raman shifts (that is, ∼ 219, 283 and 326 cm −1 ) are also associated with the phonon modes in M-MoS 2 . S-MoS 2 exhibits typical Raman shifts of ∼ 378 and 404 cm −1 for E 1 2g and A 1g , respectively, which are substantially different from those of M-MoS 2 . Figure 1: Morphology of M-MoS 2 and phase identification of M-MoS 2 and S-MoS 2 . ( a ) SEM image of M-MoS 2 showing the nanosheet structures. Scale bar, 100 nm. ( b ) Raman shift of M-MoS 2 and S-MoS 2 . ( c , d ) High-resolution X-ray photoelectron spectroscopy (XPS) spectra of Mo 3 d ( c ) and S 2 p ( d ) for M-MoS 2 and S-MoS 2 . Full size image The phase identification of the synthesized M-MoS 2 and S-MoS 2 was further studied using X-ray photoelectron spectroscopy and the results are shown in Fig. 1c,d . The Mo 3 d spectra consist of peaks located at approximately 228.7 and 231.8 eV, which correspond to the 3d 5/2 and 3 d 3/2 components, respectively, of Mo 4+ in M-MoS 2 . However, the Mo 3 d peaks of the M-MoS 2 samples also exhibit weak shoulders at the positions as those in S-MoS 2 due to the transformation of M-MoS 2 in vacuum and X-ray illumination. The details for the peak deconvolution are provided in Supplementary Fig. 3 and Supplementary Note 1 . The Mo 3 d peaks of M-MoS 2 shifted to lower binding energies by ∼ 1 eV with respect to the corresponding peaks in S-MoS 2 . This result is consistent with the previously obtained relaxation energy of 1 eV for M-MoS 2 derived from S-MoS 2 (refs 20 , 21 ). Similarly, the S 2 p peaks of M-MoS 2 were located at ∼ 161.6 and 162.7 eV, and associated with S 2 p 3/2 and 2 p 1/2 , respectively, which are also ∼ 1 eV lower than the corresponding peaks in S-MoS 2 . It is important to note that the prominent S peak located at ∼ 168 eV was absent, indicating that the sulfur atoms remain unoxidized in M-MoS 2 . However, this peak was observed in S-MoS 2 after annealing at 240 °C. 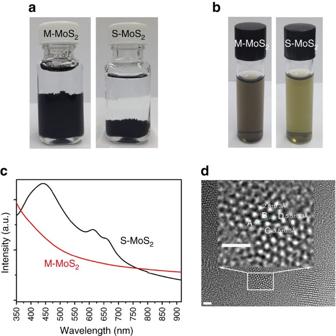Figure 2: Morphology and property of M-MoS2and S-MoS2. (a) As-prepared M-MoS2and S-MoS2in water. (b) Suspension of M-MoS2and S-MoS2in water. (c) Ultraviolet–visible absorption of M-MoS2and S-MoS2. (d) HRTEM image of M-MoS2. The region indicated by the squares is enlarged to show the atomic structure of M-MoS2. Scale bar, 1 nm. Morphologies and optical properties of MoS 2 Figure 2a shows optical images of the two types of MoS 2 dispersed in water. M-MoS 2 does not appear to exhibit bulk aggregation, whereas S-MoS 2 aggregates at the bottom of the solution. This result may be because M-MoS 2 possesses hydrophilic surfaces, whereas S-MoS 2 possesses relatively hydrophobic surfaces [5] , [22] . After sonication, both M-MoS 2 and S-MoS 2 can uniformly disperse in water ( Fig. 2b ). However, M-MoS 2 was grey colour, whereas S-MoS 2 was green colour. These colours were associated with their optical properties, which were confirmed by optical absorption spectroscopy. Figure 2c shows the ultraviolet–visible absorption spectra of M-MoS 2 and S-MoS 2 in water. Two typical absorption peaks located at 613 and 660 nm were observed for S-MoS 2 and these peaks are associated with the energy split from the valence band spin–orbital coupling in S-MoS 2 with large lateral dimensions [23] . In addition, another optical absorption band located at ∼ 442 nm was observed. This band most probably results from the quantum effect of smaller lateral-sized S-MoS 2 nanosheets. The absorption spectrum of M-MoS 2 has no salient absorption bands but a monotonic change that is indicative of its metallic property. Figure 2: Morphology and property of M-MoS 2 and S-MoS 2 . ( a ) As-prepared M-MoS 2 and S-MoS 2 in water. ( b ) Suspension of M-MoS 2 and S-MoS 2 in water. ( c ) Ultraviolet–visible absorption of M-MoS 2 and S-MoS 2 . ( d ) HRTEM image of M-MoS 2 . The region indicated by the squares is enlarged to show the atomic structure of M-MoS 2 . Scale bar, 1 nm. Full size image The atomic structure of M-MoS 2 was investigated using a high-resolution scanning transmission electron microscope (HRTEM) at different magnifications ( Supplementary Fig. 4 ) and the high-magnification image is shown in Fig. 2d . The hexagonal atomic arrangement of Mo indicates that each individual nanosheet consists of single crystal domains. Mo atoms on the basal plane have a Mo–Mo distance from A to D of 5.5±0.3 Å, A to B of 2.8±0.3 Å and A to C of 3.5±0.3 Å. However, the crystal lattice may convert into an amorphous structure under the high-energy electron beam of TEM as observed by Lukowski et al . [2] . Stability of the M-MoS 2 The as-prepared M-MoS 2 nanosheets in water exhibited good stability over time. We believe that the high purity of M-MoS 2 plays an important role in its stability. 1T-MoS 2 (metallic phase), which was derived from 2H-MoS 2 (semiconductor phase), consists of electronic heterostructures of 2H-MoS 2 and 1T-MoS 2 in individual layers of MoS 2 (ref. 9 ). The coexistence of semiconductor MoS 2 with a metallic phase in a single layer resulted in an expedited transformation of 1T back to 2H MoS 2 . Therefore, the structure was reported to be stable for 12 days with the observation of the 2H structure in water for chemically exfoliated MoS 2 (ref. 12 ). The samples obtained in this study were stored in water for more than 90 days at room temperature and no obvious change in the Raman shift was observed ( Fig. 3a ). The characteristic peaks of the stored M-MoS 2 were similar to those observed for the freshly prepared samples. This observation indicates that the as-prepared M-MoS 2 was highly stable in water. It is important to note that a traceable transformation of M-MoS 2 to S-MoS 2 may occur, as suggested by the very weak shoulder at 374 cm −1 . The pure metallic phase in the individual layers contributes to the stability of the material. A comparison of the Raman spectra of M-MoS 2 stored under different conditions and S-MoS 2 is shown in Supplementary Fig. 5 . 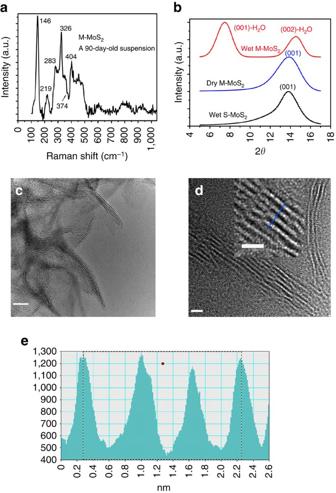Figure 3: Raman and structural characterization to investigate the stability of M-MoS2. (a) Raman shift of M-MoS2stored for 90 days at room temperature. (b) XRD patterns of wet M-MoS2, dry M-MoS2and wet S-MoS2. (c) Low-resolution TEM image of M-MoS2. Scale bar, 10 nm. (d) HRTEM image of M-MoS2. The region indicated by the square is enlarged to show the layered structure of M-MoS2. Scale bar, 2 nm. (e) Line scan of the HRTEM image indicated by the blue line ind, indicating a layer-to-layer spacing of 0.65 nm. Figure 3: Raman and structural characterization to investigate the stability of M-MoS 2 . ( a ) Raman shift of M-MoS 2 stored for 90 days at room temperature. ( b ) XRD patterns of wet M-MoS 2 , dry M-MoS 2 and wet S-MoS 2 . ( c ) Low-resolution TEM image of M-MoS 2 . Scale bar, 10 nm. ( d ) HRTEM image of M-MoS 2 . The region indicated by the square is enlarged to show the layered structure of M-MoS 2 . Scale bar, 2 nm. ( e ) Line scan of the HRTEM image indicated by the blue line in d , indicating a layer-to-layer spacing of 0.65 nm. Full size image Another possible stability mechanism may arise from the monolayer of water molecules that was adsorbed on both sides of the M-MoS 2 nanosheets. This layer prevents aggregation and stacking, and maintains the octahedral structure in M-MoS 2 . The existence of the water molecule layer was confirmed by XRD measurements ( Fig. 3b ). The peak at 7.5°, which corresponds to a spacing of 11.8 Å, was identified as (001)-H 2 O for M-MoS 2 -H 2 O, which contains a bilayer of water molecules between the adjacent layers of MoS 2 nanosheets [24] . As the layer thickness of MoS 2 was ∼ 6.2 Å and the thickness of a monolayer of water was 2.8 Å, the total thickness of a MoS 2 layer surrounded by a water bilayer would be 11.8 Å. This result was previously confirmed by XRD [25] . The peak located at 14.6° was assigned to the second-order reflection of M-MoS 2 -H 2 O. XRD was also performed on the M-MoS 2 nanosheets after they were dried for 24 h in a vacuum chamber at a pressure of 6 mTorr. The XRD pattern of the dried M-MoS 2 is similar to that of S-MoS 2 with a peak at 13.88° ( Fig. 3b ), which corresponds to the stacked M-MoS 2 multilayers. This result suggests that the spacing between the Mo planes for M-MoS 2 was 6.4±0.1 Å. This spacing is larger than that of bulk MoS 2 (that is, 6.15 Å). The diffraction peak at 7.5° disappeared due to desorption of the water molecules on the nanosheet surfaces. The TEM and HRTEM images indicate that M-MoS 2 was composed of single-layer or several-layer structures ( Fig. 3c,d ). The lattice fringe spacing of M-MoS 2 was measured to be 1.97 nm for a four-layer nanosheet, which produced a Mo–Mo spacing of 6.5±0.1 Å ( Fig. 3e ). This result is consistent with the value obtained from the XRD measurements. The increased interlayer spacing in M-MoS 2 may contribute to its stability due to the weakened S–S van der Waals interactions and reduced restacking probability. M-MoS 2 contained adsorbed water molecules, which was confirmed by XRD measurements. However, this phenomenon was not observed in S-MoS 2 nanostructures. This difference between the two phases of MoS 2 reflects the different surface properties (that is, M-MoS 2 is hydrophilic, whereas S-MoS 2 is hydrophobic). These properties are determined by the atomic structures of M-MoS 2 and S-MoS 2 . The Mo atom in M-MoS 2 is located in an octahedral S coordination, whereas the Mo atom in S-MoS 2 coordinated by six S atoms in a trigonal prismatic arrangement with S acting as a hydrophobic site and Mo serving as a hydrophilic site [26] . These different surface properties were also observed regardless of whether they were dispersed in water or deposited as thin films on substrates ( Supplementary Fig. 6 ). Contact angle measurements were conducted on both the M-MoS 2 and S-MoS 2 films. A contact angle of 25° was observed for M-MoS 2 and an angle of 118° was determined for S-MoS 2 , confirming the highly hydrophilic surface of M-MoS 2 . The details are provided in Supplementary Fig. 7 . Metallic phase MoS 2 for HER The different surface properties, atomic structure and morphology of M-MoS 2 and S-MoS 2 on substrates led to significant differences in the HER. Hydrogen production measurements were conducted for the M-MoS 2 and S-MoS 2 nanosheets deposited on glassy carbon electrodes using a three-electrode cell in a 0.5-M sulfuric acid electrolyte. 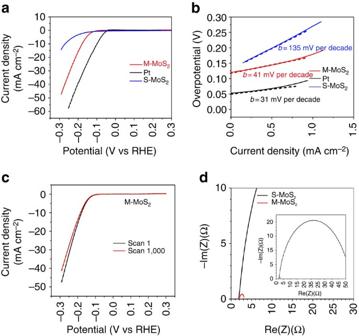Figure 4: HER activity of the synthesized MoS2nanosheets. (a) Polarization curves of the M-MoS2and S-MoS2nanosheets. (b) Corresponding Tafel plots obtained from the polarization curves. The Tafel slopes were∼41 and∼135 mV per decade for M-MoS2and S-MoS2, respectively. (c) Polarization curves of the M-MoS2nanosheets after 1 and 1,000 cycles of continuous operation. (d) Nyquist plots of M-MoS2and S-MoS2. Figure 4a,b show the polarization curves and corresponding Tafel plots of the M-MoS 2 and S-MoS 2 nanosheets compared with those of Pt. It is important to note that the Tafel plot employs a logarithmic current density axis. A low potential of −175 mV at a current density of 10 mA cm −2 and a Tafel slope of 41 mV per decade were obtained for M-MoS 2 . This observed potential for hydrogen production represents the lowest value among the reported experimental data for the use of only MoS 2 materials. The long-term stability of the M-MoS 2 electrode for the HER was investigated. After 1,000 cycles of continuous operation, the exfoliated MoS 2 nanosheets exhibited <12% decay in the electrocatalytic current density ( Fig. 4c ). The advantage of using M-MoS 2 nanosheets becomes more apparent through electrochemical impedance spectroscopy analysis. The electrochemical impedance spectroscopy was performed under the HER conditions. The Nyquist plots are shown in Fig. 4d and revealed a dramatically decreased charge transfer resistance for the M-MoS 2 nanosheets ( ∼ 1 Ω) relative to the S-MoS 2 nanosheets ( ∼ 50 Ω). Furthermore, we measured the resistivity of the M-MoS 2 (300 nm thick) and S-MoS 2 (340 nm thick) films using a four-probe method under ambient conditions. The sheet resistances are 1.61 × 10 4 Ω/□ for M-MoS 2 and 2.26 × 10 9 Ω/□ for S-MoS 2 , which correspond to a resistivity of 0.482 Ω·cm for M-MoS 2 and 7.68 × 10 4 Ω·cm for S-MoS 2 . This result indicates that M-MoS 2 has a conductivity that is five orders of magnitude higher than that of S-MoS 2 . Figure 4: HER activity of the synthesized MoS 2 nanosheets. ( a ) Polarization curves of the M-MoS 2 and S-MoS 2 nanosheets. ( b ) Corresponding Tafel plots obtained from the polarization curves. The Tafel slopes were ∼ 41 and ∼ 135 mV per decade for M-MoS 2 and S-MoS 2 , respectively. ( c ) Polarization curves of the M-MoS 2 nanosheets after 1 and 1,000 cycles of continuous operation. ( d ) Nyquist plots of M-MoS 2 and S-MoS 2 . Full size image It is important to note that the growth of M-MoS 2 and the HER measurements are highly reproducible. The growth process of M-MoS 2 failed only once in 96 trials. The failure was caused by washing the autoclave with HNO 3 and we believe that a trace amount of residual HNO 3 may have oxidized the products via different chemical reactions. The autoclave was typically cleaned by sonication in water. We have performed the HER 62 times using our synthesized M-MoS 2 and all of the trials yielded results similar to those shown in Fig. 4a,b . The exceptional performance of M-MoS 2 for hydrogen production may be due to the high purity, dense active sites, good conductivity and excellent hydrophilic property of M-MoS 2 . By contrast, S-MoS 2 exhibited little HER activity with a potential of −274 mV at 10 mA cm −2 and a Tafel slope of 135 mV per decade. The poor performance of S-MoS 2 in the HER was due to few active sites, aggregation and its hydrophobic surface. The exchange current density of M-MoS 2 , S-MoS 2 and Pt is discussed in Supplementary Discussion . Although M-MoS 2 still lags behind Pt, improvement in the HER activity can be accomplished by enhancing the conductivity of the nanoscale M-MoS 2 . Therefore, metallic MoS 2 exhibits great potential for use as a replacement for Pt in the HER as a low-cost and highly active catalyst for practical applications. The mechanism underlying the formation of the stable metallic phase of MoS 2 is directly associated with the weak reducer urea, which can precisely and effectively reduce MoO 3 to M-MoS 2 as shown in equation (1). The absence of a urea reducer while maintaining other growth conditions would result in a product dominated by amorphous MoS 3 , as shown in equation (2) (see Supplementary Methods and Supplementary Fig. 8 ). Other reducers, such as hydrazine, reduce MoO 3 to S-MoS 2 only due to the relatively strong electron donating ability of hydrazine. During the synthesis of M-MoS 2 , the three most important factors are solvent, pH and temperature. First, water serves as a solvent and is adsorbed on the surface of M-MoS 2 to form a water molecular layer that prevents layer stacking. When an organic solvent, such as ethanol or dimethylformamide, was added to the reaction, no desirable product was produced (see the Supplementary Methods and Supplementary Fig. 9 ). No solid product was found in the autoclave when a 1:1 ratio of water to ethanol was used. Second, the pH controls the steric structure of the starting materials and the formation of M-MoS 2 . When the pH value was ≤4, the octahedral coordination of MoO 3 can be maintained, which may lead to the formation of M-MoS 2 . At higher pH values (pH 8) achieved through the addition of ammonia, the MoO 3 structure converts into MoO 4 2− tetrahedral centres. This change causes the reaction to yield no desirable products. Third, the temperature also plays a key role in the formation of M-MoS 2 . In this study, pure M-MoS 2 was obtained at 200 °C and S-MoS 2 was formed at 240 °C in the reaction listed in equation (3). Based on these discussions, the metastable M-MoS 2 intermediate can be formed and stabilized in a pressurized hydrothermal process with a suitable reducer and temperature. The proposed mechanism involves the formation of a crystal phase of M-MoS 2 from amorphous clustered MoS 3 with S 2 − edge bonds reduced by urea. In fact, many investigations have revealed the structural evolution from MoS 3 to S-MoS 2 without the MoS 2 metallic phase during the evolution process [27] , [28] , [29] . We believe that the high temperature and strong reducer used in the previous studies may have only resulted in the formation of semiconductor MoS 2 . This result was also confirmed in this study, because only S-MoS 2 was obtained when the temperature was increased to 240 °C. The evolution process for the formation of M-MoS 2 is shown in Fig. 5 , which illustrates the growth of MoS 3 from one cluster to two and finally to a nanosheet. The central part possesses the structure of M-MoS 2 and the S 2 − bond on the edge can be removed by urea to continue the growth to form a single layer of M-MoS 2 (ref. 30 ). A control experiment was carried out by stopping the growth after 90 min, which resulted in a mixture of MoS 3 and M-MoS 2 in the solution. The existence of MoS 3 and its corresponding peak at 120 cm −1 peak was confirmed by Raman spectroscopy [31] . Furthermore, a Raman band located at 548 cm −1 , which was due to the S 2 − stretching vibration in MoS 3 , was observed. Energy dispersive X-ray spectroscopy measurements indicate a ratio of 1:3 for Mo and S (See Supplementary Fig. 10b ). The Mo–Mo vibration mode at 146 cm −1 starts to appear and become more prominent as growth time increased, indicating the transformation of MoS 3 to M-MoS 2 (see Supplementary Fig. 10c ). After continuing the reaction for 6 h, only M-MoS 2 was observed in the product. At this point, the Raman peak located at 120 cm −1 disappeared and the intensity of the 146 cm −1 peak reached its maximum. This result indicates the complete conversion of MoS 3 to M-MoS 2 . 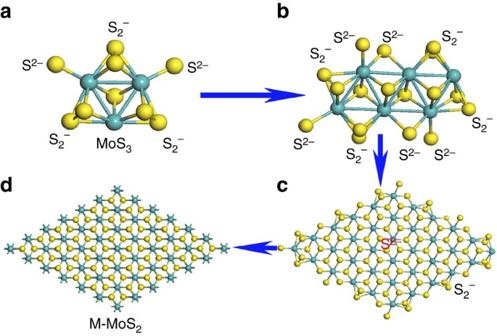Figure 5: Schematic illustrations of the evolution process of M-MoS2from MoS3. (a) One MoS3cluster with S2−and S2−. (b) Combination of two MoS3clusters with the breaking of S2−. (c) Several MoS3cluster forming MoS2with S2−in the centre and MoS3with S2−at the edge. (d) Stable M-MoS2crystal structure. Figure 5: Schematic illustrations of the evolution process of M-MoS 2 from MoS 3 . ( a ) One MoS 3 cluster with S 2− and S 2 − . ( b ) Combination of two MoS 3 clusters with the breaking of S 2 − . ( c ) Several MoS 3 cluster forming MoS 2 with S 2− in the centre and MoS 3 with S 2 − at the edge. ( d ) Stable M-MoS 2 crystal structure. Full size image A hydrothermal process has been used to grow S-MoS 2 . To the best of our knowledge, the preparation of M-MoS 2 using a hydrothermal method has not been previously reported. We believe that the growth conditions used in this study play a key role in the formation and stabilization of M-MoS 2 . M-MoS 2 is an unstable phase that can easily transform to S-MoS 2 . Therefore, the octahedral coordination of M-MoS 2 must be maintained during deposition. For this reason, we used MoO 3 as the starting material, because it possesses the same octahedral structure as M-MoS 2 . The metallic phase can be obtained when the crystal structure can be maintained during the conversion process from MoO 3 to MoS 2 . Urea, which is a weak reducer, is able to maintain the crystal structure at a low pH value and optimum temperature (200 °C) for hydrothermal growth. As mentioned in the previous sections, only S-MoS 2 was obtained at a higher growth temperature of 240 °C, because the octahedral structure of M-MoS 2 cannot be maintained under the growth conditions used. Once the M-MoS 2 nanosheets were formed at 200 °C, the adsorption of water molecules on their surfaces due to the hydrophilic nature of the surface provides an environment to maintain the octahedral structure and preventing restacking of the layers. Therefore, M-MoS 2 can be stored in water for several months without significant transition to S-MoS 2 . However, once M-MoS 2 is removed from water and dried in a vacuum, it will slowly convert to S-MoS 2 . This observation indicates that the stability of M-MoS 2 is dependent on the environment. Although this study was focused on the influence of water, the environmental stability of M-MoS 2 under other conditions, such as different gases and solutions other than water, should be considered in future investigations. In conclusion, highly pure and stable M-MoS 2 nanosheets were synthesized in solution using a rational and controllable approach. A unique Raman peak located at 146 cm −1 due to M-MoS 2 was experimentally observed, which confirms the theoretical prediction. A growth mechanism was proposed and is supported by the experimental data. Excellent activity of M-MoS 2 for the HER was achieved and the material has the potential to replace Pt in practical applications. These results provide opportunities for studying the metallic phase of MoS 2 , which has potential technological applications in renewable energy, energy storage and heterogeneous catalysis. Preparation of M-MoS 2 and S-MoS 2 MoO 3 powder (CAS number is 1311-27-5) and urea (CAS number is 57-13-6) were purchased from the Sigma-Aldrich Company. Thioacetamide (CAS number is 62-55-5) was purchased from the Fisher Scientific Company. The autoclave (model number 4749) was ordered from the Parr Instrument Company. Twelve milligrams of MoO 3 , 14 mg of thioacetamide and 0.12 g of urea were dissolved in 10 ml of deionized water and stirred for 2 h. Then, the solution was placed in an autoclave and loaded into a furnace (from MTI), which has been heated to 200 °C. The temperature of the oven was maintained at 200 °C for 12 h. Next, the reaction was terminated by rapidly cooling the solution to room temperature by removing the autoclave from the oven. The prepared M-MoS 2 was collected and washed with deionized water several times, followed by storage in deionized water before use. The same procedure was used to synthesize S-MoS 2 at 240 °C. Two-dimensional nanosheets were observed and no significant difference was observed between M-Mo 2 and S-MoS 2 based on their nanoscale morphology. Ultraviolet–visible–infrared spectroscopy Ultraviolet–visible–infrared absorption spectroscopy of the M-MoS 2 and S-MoS 2 dispersions in water were recorded using a Perkin Elmer Lambda 25 spectrophotometer. TEM observations TEM and HRTEM images and electron diffraction were performed on a FEI Tecnai G2 F20 S-Twin microscope operated at an accelerating voltage of up to 200 kV. The TEM samples were prepared by sonication at 500 W for ∼ 5 min and 25 μl of the supernatant were dropped onto holey carbon grids. SEM observations The SEM images were obtained using a field-emission gun SEM (Quanta 400 FEG FEI). The samples were dispersed in water and then dropped onto the Si/SiO 2 substrates. X-ray photoelectron spectroscopy X-ray photoelectron spectroscopy was conducted using an Axis Ultra DLD (Kratos) system. The vacuum of the chamber was 1 × 10 −9 Torr. A monochromatic aluminum K α source with a source power of 150 W (15 kV × 10 mA) was used. The pass energy was 160 eV for wide scans and 40 eV for narrow scans. Raman spectroscopy Raman spectroscopy was performed using a LabRam HR800 UV NIR and 532-nm laser excitation with working distances on a × 50 lens. The Raman spectra of M-MoS 2 and S-MoS 2 were recorded by depositing the samples on silicon substrates. XRD patterns The XRD patterns of M-MoS 2 and S-MoS 2 were recorded for two theta values ranging from 4° to 18°, to characterize the interlayer spacing. The characterization was performed on a Bruker AXS-D8 Advance powder X-ray diffractometer using Cu/Ka radiation ( λ =1.5406 Å) with a step size of 0.02° and a dwell time of 3.0 s. Electrocatalytic hydrogen evolution The electrochemical measurements were performed using a three-electrode electrochemical station (Gamry Instruments). All of the measurements were performed in a solution consisting of 50 ml of a 0.5-M H 2 SO 4 electrolyte prepared using 18 M deionized water purged with H 2 gas (99.999%). The MoS 2 suspension in water was dropped onto glassy carbon as the working electrode. All of the working electrodes were prepared using the MoS 2 solutions. The solution concentrations of M-MoS 2 and S-MoS 2 were ∼ 0.3 mg ml −1 and ∼ 0.4 mg ml −1 , respectively, in water. The diameter of the glass carbon electrode was 0.3 cm and the area was ∼ 0.07 cm 2 . The amount of deposited catalyst on the electrode was ∼ 43 μg cm −2 for M-MoS 2 and 114 μg cm −2 for S-MoS 2 . Platinum foil was used as the counter electrode and a saturated calomel was used as the reference electrode. The reversible hydrogen electrode was calibrated using platinum as both the working and counter electrodes to +0.3 V versus the saturated calomel reference electrode. The performance of the hydrogen evolution catalyst was measured using linear sweep voltammetry from +0.3 to −0.3 V versus reversible hydrogen electrode with a scan rate of 5 mV s −1 . How to cite this article : Geng, X. et al . Pure and stable metallic phase molybdenum disulfide nanosheets for hydrogen evolution reaction. Nat. Commun. 7:10672 doi: 10.1038/ncomms10672 (2016).